A new method to position and functionalize metal-organic framework crystals With controlled nanometre-sized pores and surface areas of thousands of square metres per gram, metal-organic frameworks (MOFs) may have an integral role in future catalysis, filtration and sensing applications. In general, for MOF-based device fabrication, well-organized or patterned MOF growth is required, and thus conventional synthetic routes are not suitable. Moreover, to expand their applicability, the introduction of additional functionality into MOFs is desirable. Here, we explore the use of nanostructured poly-hydrate zinc phosphate (α-hopeite) microparticles as nucleation seeds for MOFs that simultaneously address all these issues. Affording spatial control of nucleation and significantly accelerating MOF growth, these α-hopeite microparticles are found to act as nucleation agents both in solution and on solid surfaces. In addition, the introduction of functional nanoparticles (metallic, semiconducting, polymeric) into these nucleating seeds translates directly to the fabrication of functional MOFs suitable for molecular size-selective applications. Ordered nanoporous systems with a large and accessible surface area are desirable in many applications, which require controlled molecular transport properties [1] . Metal-organic frameworks (MOFs) possess high surface areas [2] , adaptable surface chemistries, pore sizes [3] and structures [4] that make them leading candidates to separate [5] , capture [6] , store [7] , deliver [8] , transport [9] , sense [10] and catalyse [11] molecules. MOFs (or coordination polymers with permanent porosity [4] ) also have exciting potential as light-weight molecular selective sieves, because of their extremely high surface areas, low density, interconnected cavities and very narrow pore size distributions [12] . Some frameworks are also adaptive materials which respond to external stimuli (for example, light, electrical field, presence of particular chemical species), promising new advanced practical applications [6] , [10] , [13] . To gain adoption in devices, a straightforward method to deposit MOFs onto chemically differing substrates must first be developed, preferably avoiding substrate functionalization protocols. In addition to permitting controlled MOF growth at specific locations on planar substrates, this method must also be adaptable to more complex two-dimensional (2D) and three-dimensional (3D) surface morphologies. Achieving such facile deposition and growth requires a new level of control in the field of MOF synthesis. Further to spatial control of MOF growth, full exploitation of their properties in next generation sensing, separation, catalysis and delivery devices may require the introduction of extrinsic functionality (for example, magnetism, luminescence and so on). Ideally, the functionality would reside within the core of the MOF so that the favourable selective barrier properties provided by the framework could impart molecule-specificity to the devices. Incorporation of functional species in MOFs has to date been demonstrated through post-impregnation mostly of metal nanospecies by chemical vapour deposition [14] and one-pot synthesis (adding either the functional species [15] or its precursors [16] directly into the MOF growing medium). Both of these approaches cause the doping species to grow indiscriminately inside the MOF cavities and on the MOF outer surface. The resulting lack of spatial control of the functional components within the MOF crystals compromises the molecular selectivity of the final composite. Here, we present a novel and straightforward method ( Fig. 1 ) to simultaneously achieve MOF positioning and functionalization. The method is based on our discovery that a class of nanostructured α-hopeite microparticles shows an exceptional ability to nucleate MOFs. These microparticles are used as seeds for growing MOFs in solution ( Fig. 1a ), on any flat surface ( Fig. 1b ) and on complex 2D/3D surface morphologies ( Fig. 1c ). In addition, the introduction of active species (either metal, semiconductor or polymer nanoparticles) directly into the framework via the α-hopeite microparticles, permits functionalization solely within the framework core, and not on its outer surface ( Fig. 1d ). Unlike the previously reported studies on functionalization of MOFs, the unprecedented spatial control that is offered through our method enables various functionalities to be easily included within each MOF crystal, without compromising the size-selective properties of the framework. A single crack or pinhole could make the putative sieving ineffective with respect to subsequent selective chemical reactivity; however, the MOF composites described here are free of such defects. The method allows for the MOF shell to behave as a molecular sieve for the encapsulated functional species ( Fig. 1e ). We focus on the archetypal MOF-5 (refs 3 , 17 ) to benchmark the use of the α-hopeite microparticles as nucleating seeds and as carriers for embedding controlled functionality. Given the peculiar resemblance of these inorganic microparticles to the desert rose mineral, we have named them as desert rose microparticles (DRMs). This report demonstrates that using DRMs to nucleate MOFs not only promotes faster MOF formation in solution but also enables controlled MOF formation on any surface chemistry and morphology. In addition, DRMs offer the unprecedented means to effectively encapsulate a range of functional nanospecies of diverse chemical nature (for example, metal, polymer, semiconductor) within MOFs. The successful coupling of the sieving effect of the MOF matrix and the preserved functionality of the embedded species opens a new route for the development of a future generation of micro-reactors for selective sensing and catalysis. 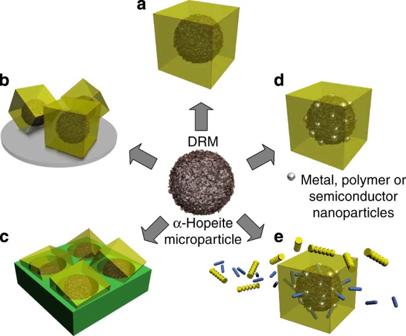Figure 1: Possibilities offered by desert rose microparticles. (a) The ceramic desert rose microparticles (DRMs, α-hopeite microparticles) enable the preparation of MOF-5 in a one-pot synthesis, reducing the crystal formation time. (b) DRMs can be used to seed MOF-5 growth on any substrate, without the need for chemical functionalization of the surface. (c) The ceramic microparticles have been combined with a lithographed surface affording spatial control of MOF growth. (d) The α-hopeite microparticles can be synthesized in the presence of functional nanoparticles, including metal (Pt and Pd), polymer (PTFE) and semiconductor (CdSe-CdS-ZnS quantum dots) nanoparticles. The functionalized DRMs can be subsequently used to grow MOF-5. One advantage of this synthesis route is the ability to embed nanoparticles solely in the core of the MOF crystals. (e) The method enables the preparation of new molecular sieves in which, depending on their size, only selected molecules can diffuse through the framework (blue molecules) accessing the functional core; diffusion is not allowed for bigger molecules (yellow molecules). With this synthesis route new devices such as selective catalysts and luminescent sensors can be prepared. Figure 1: Possibilities offered by desert rose microparticles. ( a ) The ceramic desert rose microparticles (DRMs, α-hopeite microparticles) enable the preparation of MOF-5 in a one-pot synthesis, reducing the crystal formation time. ( b ) DRMs can be used to seed MOF-5 growth on any substrate, without the need for chemical functionalization of the surface. ( c ) The ceramic microparticles have been combined with a lithographed surface affording spatial control of MOF growth. ( d ) The α-hopeite microparticles can be synthesized in the presence of functional nanoparticles, including metal (Pt and Pd), polymer (PTFE) and semiconductor (CdSe-CdS-ZnS quantum dots) nanoparticles. The functionalized DRMs can be subsequently used to grow MOF-5. One advantage of this synthesis route is the ability to embed nanoparticles solely in the core of the MOF crystals. ( e ) The method enables the preparation of new molecular sieves in which, depending on their size, only selected molecules can diffuse through the framework (blue molecules) accessing the functional core; diffusion is not allowed for bigger molecules (yellow molecules). With this synthesis route new devices such as selective catalysts and luminescent sensors can be prepared. Full size image Nucleating properties of DRMs in solution We have optimized a one-pot synthesis to grow MOF-5 through a surfactant assisted (Pluronic F-127) method. Once added to a traditional MOF-5 precursor solution, this particular surfactant coordinates the Zn 2+ ions [18] , [19] and contemporaneously provides an abundant source of phosphate (see Supplementary Fig. S1 ). These factors enable the rapid and iso-directional formation of inorganic poly-hydrate zinc phosphate nanoflaked microparticles (DRMs, see Fig. 2a ) within the framework precursor solution. The chemical and morphological characterization of the DRMs is presented in Supplementary Figures S2, S3 and Supplementary Table S1 . The nanostructured microparticles form within the first minute of reaction inside the cloudy surfactant suspension that constitutes the MOF-5 precursor solution, and in the following 3 h the DRMs grow up to tens of microns. As the DRM formation precedes the growth of MOF-5, DRMs can effectively act as heterogeneous nucleation seeds for the framework crystals ( Fig. 2b–d and Supplementary Fig. S4 ). 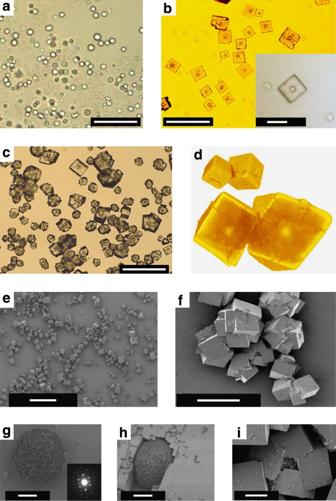Figure 2: Desert rose microparticles and their nucleating effect. (a–c) Optical microscope images of the desert rose microparticles (DRMs) and MOF-5 crystals formed using DRMs as seeds. (a) DRMs formed in the MOF growing medium containing Pluronic F-127 after 3 h reaction at 95 °C (scale bar, 100 μm). The picture shows a group of DRMs that grew within the suspended cloud of Pluronic F-127; the cloud is also visible in the image. The average size of the DRMs is in the tens of microns range. The picture was taken of a drop of solution extracted from the mother batch and dropped directly on a glass microscope slide. (b) MOF-5 crystals formed around the DRMs. The image was taken of a drop of solution extracted after 8 h reaction at 95 °C (scale bar, 200 μm, inset scale bar, 50 μm). (c) Two-step heating synthesis resulting in multicrystalline growth on each DRM (scale bar, 200 μm). (d) X-ray microtomography performed on two cubic crystals of MOF-5 nucleated around two DRMs. The small images on the top-left are the measured tomography of the crystals' exterior surfaces. The main image is a cross-section of the cubic crystals. The image was obtained slicing the 3D tomographs along a section plane, which intersects both of the crystal centres and is perpendicular to the observer's view. The exposed section demonstrates that the DRMs are sitting in the geometric centre of the cubic crystals. (e–i) SEM images of the MOF-5 crystals grown with the assistance of the DRMs. (e) Overview of cubic MOF-5 crystals resulting from the one-pot synthesis (scale bar, 500 μm). (f) MOF-5 crystals grown using the two-step synthesis (scale bar, 50 μm). (g) Close-up of a DRM particle. This image reveals the faceted features of the DRMs surface (scale bar, 5 μm). The inset of the figure shows the electron diffraction pattern of the DRMs, indexed as α-hopeite. (h) DRMs partially embedded in the MOF structure (one-pot synthesis). Scale bar, 5 μm. (i) DRMs almost completely embedded in the MOF structure (two-step synthesis). Scale bar, 10 μm. Figure 2: Desert rose microparticles and their nucleating effect. ( a – c ) Optical microscope images of the desert rose microparticles (DRMs) and MOF-5 crystals formed using DRMs as seeds. ( a ) DRMs formed in the MOF growing medium containing Pluronic F-127 after 3 h reaction at 95 °C (scale bar, 100 μm). The picture shows a group of DRMs that grew within the suspended cloud of Pluronic F-127; the cloud is also visible in the image. The average size of the DRMs is in the tens of microns range. The picture was taken of a drop of solution extracted from the mother batch and dropped directly on a glass microscope slide. ( b ) MOF-5 crystals formed around the DRMs. The image was taken of a drop of solution extracted after 8 h reaction at 95 °C (scale bar, 200 μm, inset scale bar, 50 μm). ( c ) Two-step heating synthesis resulting in multicrystalline growth on each DRM (scale bar, 200 μm). ( d ) X-ray microtomography performed on two cubic crystals of MOF-5 nucleated around two DRMs. The small images on the top-left are the measured tomography of the crystals' exterior surfaces. The main image is a cross-section of the cubic crystals. The image was obtained slicing the 3D tomographs along a section plane, which intersects both of the crystal centres and is perpendicular to the observer's view. The exposed section demonstrates that the DRMs are sitting in the geometric centre of the cubic crystals. ( e – i ) SEM images of the MOF-5 crystals grown with the assistance of the DRMs. ( e ) Overview of cubic MOF-5 crystals resulting from the one-pot synthesis (scale bar, 500 μm). ( f ) MOF-5 crystals grown using the two-step synthesis (scale bar, 50 μm). ( g ) Close-up of a DRM particle. This image reveals the faceted features of the DRMs surface (scale bar, 5 μm). The inset of the figure shows the electron diffraction pattern of the DRMs, indexed as α-hopeite. ( h ) DRMs partially embedded in the MOF structure (one-pot synthesis). Scale bar, 5 μm. ( i ) DRMs almost completely embedded in the MOF structure (two-step synthesis). Scale bar, 10 μm. Full size image The micron dimensions of both the DRMs and the MOF-5 crystals ensure that optical microscopy is a convenient tool to study the nucleation and growth processes within our surfactant assisted growth solution. During the first 3 h of reaction, the only micron-sized species to form within the surfactant suspension are the α-hopeite DRMs of Figure 2a . After 3 h, heterogeneous nucleation of MOF-5 takes place on the nanometre-sized flakes of the DRMs to form cubic crystallites ( Supplementary Figs S5–S8 ). Prolonging this growth time allows single crystal ( Fig. 2b ) or multifaceted ( Fig. 2c ) MOF-5 crystallites to develop, with sizes as large as 100 μm. We observed that the controlled MOF-5 growth through heterogeneous crystallization reduces the MOF-5 synthesis time by 70% when compared with conventional solvothermal methods. Statistical analysis of individual MOF-5 crystals indicates that on average 96% contain one α-hopeite DRM when synthesized in dimethyl formamide (DMF; Fig. 2b ). By adopting an optimized two-step thermal process, up to 98% of these DRMs generate a crystal of MOF-5 ( Fig. 2c ). X-ray microtomography analysis ( Fig. 2d ) confirms that the embedded microparticles sit at the centre of each cubic crystal. The microparticle spheres have a density similar to the surrounding coordination polymer and possess a lower density shell. The resulting crystals appear in the SEM images of Figure 2e,f . Scanning electron microscopy of MOF-5 synthesized using the surfactant-directed method reveals that the spherical shape of the α-hopeite DRMs is produced by the arrangement of multiple 150–200 nm thick interpenetrating plates ( Fig. 2g ). Furthermore, it can be understood from Figure 2h,i that the microparticles that nucleate and promote growth of the MOF-5 crystals are progressively embedded deeper within the framework during the growth stage. Spatial control of MOF growth During a single-pot synthesis, α-hopeite DRMs can be isolated before MOF-5 nucleates, and consequently re-dispersed into a variety of solvents as exogenous nucleation seeds. When incubated in a fresh N,N- diethyl formamide (DEF)-based MOF-5 growth medium, a significant improvement in crystal quality can be achieved ( Supplementary Figs S9, S10 ). The use of the nucleating agents in this case more than doubles the crystal growth rate compared with control samples. The seeded nucleation mechanism for the growth of MOF-5 can be adapted directly to solid substrates. This feature is demonstrated for α-hopeite DRMs deposited directly onto an alumina or silicon substrate ( Fig. 3a ). 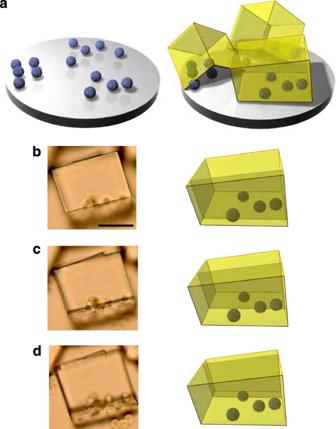Figure 3: Desert rose microparticle assisted growth of MOF-5 on a flat surface. (a) Schematic representation of DRMs used for the nucleation of MOF-5 on a silicon surface. DRMs extracted from the growing medium are first dried on a substrate, which is subsequently immersed into a fresh DEF-based MOF-5 precursor solution. MOF-5 crystals are observed to form on the deposited bed of DRMs in the form of truncated cubes because of the flat surface of the support. (b–d) Optical microscope images of a single truncated MOF-5 crystal grown on a bed of DRMs (scale bar, 100 μm). The three images were taken on the same crystal at different microscope focal planes. Next to each image, a 3D schematic illustrates the focal plane position related to the corresponding image. As shown in Figure 3b–d , immersion of this substrate into a fresh DEF-based MOF-5 precursor solution results in crystallite growth of the framework exclusively from the microparticles (a continuous layer of crystals grown on the α-hopeite seeds is shown in Supplementary Fig. S11 ). Optical imaging through the focal plane of the frameworks reveals that several α-hopeite DRMs can be detected within the crystals. The existence of embedded microparticles and the truncated shape of the otherwise cubic crystals suggest a heterogeneous nucleation mechanism [20] . Figure 3: Desert rose microparticle assisted growth of MOF-5 on a flat surface. ( a ) Schematic representation of DRMs used for the nucleation of MOF-5 on a silicon surface. DRMs extracted from the growing medium are first dried on a substrate, which is subsequently immersed into a fresh DEF-based MOF-5 precursor solution. MOF-5 crystals are observed to form on the deposited bed of DRMs in the form of truncated cubes because of the flat surface of the support. ( b – d ) Optical microscope images of a single truncated MOF-5 crystal grown on a bed of DRMs (scale bar, 100 μm). The three images were taken on the same crystal at different microscope focal planes. Next to each image, a 3D schematic illustrates the focal plane position related to the corresponding image. Full size image In a subsequent experiment, the DRM seeding effect was tested using a support with a complex 3D geometry ( Fig. 4a–d ). A 100-μm-thick film of commercial SU-8 resist was deposited on a silicon substrate and patterned using deep X-ray lithography, to obtain an array of high aspect ratio vertical wells (30–50 μm diameter). Under optimized conditions, an average of one DRM could be deposited per well ( Fig. 4e,f ). Immersion of the DRM infiltrated surface into a MOF-5 growth solution caused framework crystals to nucleate inside the wells ( Fig. 4g ). The crystallite sizes were found to be constrained until they had outgrown the well height, whereupon they grew freely in all directions ( Fig. 4h ). Further evolution of the system resulted in the merging of MOF crystals to form an interpenetrated crystalline structure. This structure could be detached from the silicon wafer to form a free-standing support, with the channels in the SU-8 resin occupied by MOFs. Details of the procedure and examples of MOF growth on different 3D geometries are presented in Supplementary Figures S12 and S13 . 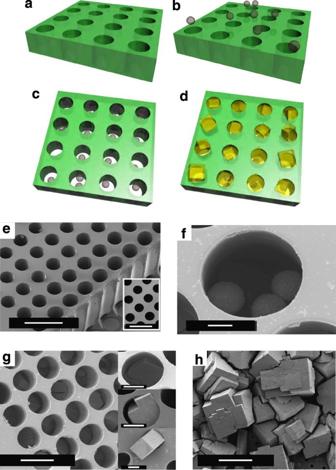Figure 4: Desert rose microparticles used for positioning MOF-5 on patterned supports. (a–d) Schematics of the procedure used to spatially drive MOF-5 formation using DRMs in pre-defined positions on a lithographed substrate. X-ray lithography was used to produce a membrane with an even distribution of wells (a) on a commercial resist (SU-8) layer previously deposited on a silicon substrate. (b) Subsequently, drops of a DRM suspension in DMF were deposited by drop-casting on the patterned substrate. (c) The substrate was vacuum dried to fill the lithographed wells with DRMs. (d) The seeded substrate was then inserted into a standard MOF-5 growing medium to induce MOF formation within the membrane holes. (e–h) SEM images showing seeding and MOF crystal growth on the lithographed substrate. (e) The SU-8 membrane obtained after the lithographic procedure. The wells have a diameter of 40 μm and a depth of 100 μm (scale bar, 100 μm). (f) DRMs located in a hole of the substrate after the drop-casting and drying processes (scale bar, 10 μm). (g) MOF-5 crystals growing within each one of the lithographed holes. The micrograph was taken after 5 h reaction time at 95 °C in the MOF-5 growing medium (scale bar, 50 μm). The insets show crystals emerging from the holes during growth (scale bar, 20 μm). (h) Substrate after 10 h reaction at 95 °C. MOF-5 crystals have grown out of the holes and appear to be interconnected with their neighbours, which is a prerequisite for the controlled formation of a continuous layer of MOF. Scale bar, 200 μm. Figure 4: Desert rose microparticles used for positioning MOF-5 on patterned supports. ( a – d ) Schematics of the procedure used to spatially drive MOF-5 formation using DRMs in pre-defined positions on a lithographed substrate. X-ray lithography was used to produce a membrane with an even distribution of wells ( a ) on a commercial resist (SU-8) layer previously deposited on a silicon substrate. ( b ) Subsequently, drops of a DRM suspension in DMF were deposited by drop-casting on the patterned substrate. ( c ) The substrate was vacuum dried to fill the lithographed wells with DRMs. ( d ) The seeded substrate was then inserted into a standard MOF-5 growing medium to induce MOF formation within the membrane holes. ( e – h ) SEM images showing seeding and MOF crystal growth on the lithographed substrate. ( e ) The SU-8 membrane obtained after the lithographic procedure. The wells have a diameter of 40 μm and a depth of 100 μm (scale bar, 100 μm). ( f ) DRMs located in a hole of the substrate after the drop-casting and drying processes (scale bar, 10 μm). ( g ) MOF-5 crystals growing within each one of the lithographed holes. The micrograph was taken after 5 h reaction time at 95 °C in the MOF-5 growing medium (scale bar, 50 μm). The insets show crystals emerging from the holes during growth (scale bar, 20 μm). ( h ) Substrate after 10 h reaction at 95 °C. MOF-5 crystals have grown out of the holes and appear to be interconnected with their neighbours, which is a prerequisite for the controlled formation of a continuous layer of MOF. Scale bar, 200 μm. Full size image Fabrication of functional framework nanocomposites By adopting a straightforward combinatorial method, the DRMs can also be doped with functional nanoparticles. We optimized a series of protocols to effectively incorporate metal (Pt and Pd), semiconductor (luminescent CdSe-CdS-ZnS quantum dots, QDs) and polymer (polytetrafluoroethylene, PTFE) nanoparticles with the DRMs. In a typical synthesis, nanoparticles of a specific functionality are introduced into the DRM growth solution. During this step, we observed that the nanoparticles spontaneously decorate the DRMs. In a first experiment, the reaction was allowed to proceed (one-pot approach) and the functionalized DRMs nucleated MOF-5 crystals directly in the same reaction batch. In a second experiment, the functionalized DRMs were isolated and inoculated into a DEF-based MOF growth medium as external seeds and produced high quality framework composites. In both the tests, the observed kinetics of MOF-5 growth showed no appreciable change compared with the synthesis without nanoparticles. In each case, the seeded MOF-5 synthesis yields framework composites containing the extrinsic functionality originating from the nanoparticles decorating the DRMs (see Methods section and Supplementary Figs S14–S19 for details). An elemental analysis of the sectioned crystals confirms signals of platinum, palladium, cadmium or fluoro species originating exclusively from the microparticles ( Fig. 5a–f ). No trace of the functional nanoparticles was recorded in the framework matrix or the framework external surface. 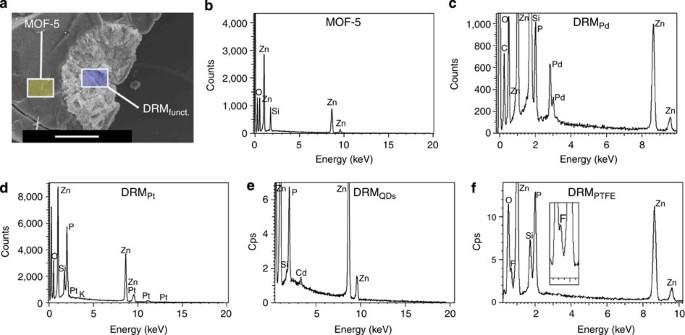Figure 5: Desert rose microparticles functionalized with functional nanoparticles. (a) SEM of a MOF-5 crystal sectioned along its median plane to expose the functionalized embedded desert rose microparticle (DRM). This MOF-5 crystal was grown around a DRM functionalized with Pd. Similar images have been obtained for each reported system involving functionalized DRMs (DRMfunct. with funct.=Pd, Pt, QDs or PTFE nanoparticles). Scale bar, 5 μm. (b) Energy dispersive X-ray analysis (EDX) of MOF-5 crystal sections. Only signals from MOF-5 constituents (C, Zn, O) are detected. The Si signal is related to the silicon wafer used as support for MOF-5 crystal analysis. (c–f) EDX of functionalized DRMs. (c) Pd functionalized DRM revealing Lα and Lβ emission from Pd atoms. (d) Pt functionalized DRM showing Lα and Lβ emissions from Pt atoms. (e) EDX of DRMs functionalized with CdSe-CdS-ZnS core-shell quantum dots revealing Lα emission of Cd only from the microsphere section. (f) Presence of a weak signal of F on the microsphere embedding PTFE nanoparticles. The experiment demonstrates the accuracy offered by the DRM approach in the control of the spatial distribution of functional species within a MOF framework. Figure 5: Desert rose microparticles functionalized with functional nanoparticles. ( a ) SEM of a MOF-5 crystal sectioned along its median plane to expose the functionalized embedded desert rose microparticle (DRM). This MOF-5 crystal was grown around a DRM functionalized with Pd. Similar images have been obtained for each reported system involving functionalized DRMs (DRM funct . with funct.=Pd, Pt, QDs or PTFE nanoparticles). Scale bar, 5 μm. ( b ) Energy dispersive X-ray analysis (EDX) of MOF-5 crystal sections. Only signals from MOF-5 constituents (C, Zn, O) are detected. The Si signal is related to the silicon wafer used as support for MOF-5 crystal analysis. ( c – f ) EDX of functionalized DRMs. ( c ) Pd functionalized DRM revealing Lα and Lβ emission from Pd atoms. ( d ) Pt functionalized DRM showing Lα and Lβ emissions from Pt atoms. ( e ) EDX of DRMs functionalized with CdSe-CdS-ZnS core-shell quantum dots revealing Lα emission of Cd only from the microsphere section. ( f ) Presence of a weak signal of F on the microsphere embedding PTFE nanoparticles. The experiment demonstrates the accuracy offered by the DRM approach in the control of the spatial distribution of functional species within a MOF framework. Full size image To demonstrate perfect encapsulation of the functional species within the MOF framework, we tested the effectiveness of the framework as a size-sieving shell. As a proof of concept, we show that the luminescent QDs/DRM/MOF-5 composites can be used to discriminate thiols of different size, thus acting as selective molecular sieve sensors. QDs that are dispersed in DEF undergo rapid quenching of the steady-state photoluminescence when thiols are injected ( Supplementary Fig. S20 ). The quenching mechanism is associated with the rapid and efficient photo-generated hole capture by surface-bound thiolates. The exact yield of luminescence quenching is directly related to the local concentration of thiol species [21] . The change in the luminescence yield of QDs that are incorporated within a MOF can therefore be used as a direct indicator of the concentration of thiol species that have diffused through the porous framework. One of the quenching thiols is a custom non-commercial copolymer, and details of its synthesis and characterization can be found in the Methods section and in Supplementary Figures S21, S22 and in Supplementary Table S2 . Luminescent MOF-5 crystals were fabricated using DRMs doped with CdSe-CdS-ZnS core-shell QDs emitting at 576 nm ( Supplementary Fig. S23 ). The resulting QDs/DRM/MOF-5 composites were loaded into DEF-filled cuvettes, and then solutions of thiols of different molecular size were injected. In situ emission spectra of the samples were recorded at 10 min intervals for times between 20 and 50 h. Equivalent experiments conducted on QDs dispersed directly in DEF show rapid and efficient luminescence quenching, regardless of the thiol molecular dimension ( Fig. 6a–c ). However, for the QDs/DRM/MOF-5 composites significant differences between the luminescence quenching results were observed depending on the size of the thiol ( Fig. 6d–f ). The smallest thiol (ethanethiol), which can readily diffuse through the MOF-5 cage, quenched 90% of the emission in about 3 h; the medium-sized thiol (2-amino-6-mercaptopurine riboside), the size of which is comparable with the dimension of MOF-5 cavities, showed a remarkably slower quenching effect (about 30% emission drop in 21 h); the biggest thiol molecule (thiol terminated copolymer n -isopropyl acrylamide/acrylic acid/ t -butyl acrylamide) did not provoke any detectable emission quenching, even after 51 h following injection. The vastly different fluorescence response of the thiols can be attributed to the sieving effect of the MOF-5 crystal, which effectively discriminates the quenching molecules by their size. Additional details can be found in the Methods section and in Supplementary Figures S24–S27 . 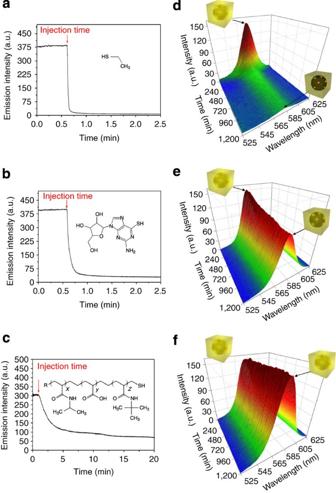Figure 6: Molecular sieving test performed with MOF-5 crystals containing desert rose microparticles functionalized with quantum dots. (a–c) Real-time emission intensity at 576 nm of quantum dots (QDs) in solution showing the quenching effect of thiols with different molecular size. (a) Using a small thiol (ethanethiol), the emission intensity drops almost instantly. (b) Using a thiol of medium size (2-amino-6-mercaptopurine riboside), a strong decrease in intensity is rapidly detected. (c) The injection of a bigger thiol (n-isopropyl acrylamide/acrylic acid/t-butyl acrylamide mercaptane) provokes a 75% decrease of the emission intensity within 15 min. Each of these thiols strongly quenched the luminescence of QDs. (d–f) Real-time luminescent spectra in the 525–625 nm range for MOF-5 crystals containing desert rose microparticles functionalized with quantum dots, that is, QDs/DRM/MOF-5 composites (details presented in the Methods section and in theSupplementary Figs S23–S27). The same thiols previously tested with the QDs in solution have been used to test the molecular sieving effect of the MOF-5 shell. (d) The small thiol (ethanethiol) quenches the luminescence of the QDs in the DRMs embedded in the MOF crystal in about 200 min. (e) The medium thiol quenches the luminescence by about 60% in 1,200 min, taking a much longer time to diffuse through the MOF. (f) The big thiol does not quench the luminescence because its large size prevents it from diffusing through the MOF to reach the QDs. (The experiment was interrupted after 50 h with no change in luminescence intensity). Figure 6: Molecular sieving test performed with MOF-5 crystals containing desert rose microparticles functionalized with quantum dots. ( a – c ) Real-time emission intensity at 576 nm of quantum dots (QDs) in solution showing the quenching effect of thiols with different molecular size. ( a ) Using a small thiol (ethanethiol), the emission intensity drops almost instantly. ( b ) Using a thiol of medium size (2-amino-6-mercaptopurine riboside), a strong decrease in intensity is rapidly detected. ( c ) The injection of a bigger thiol ( n -isopropyl acrylamide/acrylic acid/ t -butyl acrylamide mercaptane) provokes a 75% decrease of the emission intensity within 15 min. Each of these thiols strongly quenched the luminescence of QDs. ( d – f ) Real-time luminescent spectra in the 525–625 nm range for MOF-5 crystals containing desert rose microparticles functionalized with quantum dots, that is, QDs/DRM/MOF-5 composites (details presented in the Methods section and in the Supplementary Figs S23–S27 ). The same thiols previously tested with the QDs in solution have been used to test the molecular sieving effect of the MOF-5 shell. ( d ) The small thiol (ethanethiol) quenches the luminescence of the QDs in the DRMs embedded in the MOF crystal in about 200 min. ( e ) The medium thiol quenches the luminescence by about 60% in 1,200 min, taking a much longer time to diffuse through the MOF. ( f ) The big thiol does not quench the luminescence because its large size prevents it from diffusing through the MOF to reach the QDs. (The experiment was interrupted after 50 h with no change in luminescence intensity). Full size image The role played by a surfactant (Pluronic F127) in the classical solvothermal synthesis of MOF-5 has been investigated for the first time. This surfactant has been used to create a novel ceramic microparticle in which nanosized flakes are arranged to form a spherical microscopic superstructure. The unexpected windfall of these α-hopeite microparticles, here named as DRMs, is to offer an ideal combination of chemistry and morphology for MOF-5 growth. As an immediate consequence, DRMs enhance the growth rate of the framework by a factor of three compared with conventional solvothermal synthesis. The versatility of the DRMs can be extended through their isolation and then use as heterogeneous seeds to trigger MOF nucleation on either flat surfaces or 3D objects. A number of recent studies have explored a variety of protocols and patterning technologies [22] , [23] , [24] , [25] , [26] to grow MOFs in selected areas [27] , all of which have been limited to planar surfaces. To extend the 2D lithography methods for MOF growth to more complex 3D surfaces, we showed that DRMs can be used to fabricate free-standing MOF-5 forms using lithographically patterned substrates. We showed that positioning the DRMs allows for spatially controlled growth of MOF-5 and offers new routes to fabricate 2D or 3D architectures of MOF-5. With this method, there is no need for chemical functionalization of the surface because positioning the DRMs is enough to localize the framework growth. Here, we propose new routes for the simultaneous fast growth and controlled positioning of frameworks; both features are fundamental prerequisites for framework device fabrication. An additional degree of freedom offered by the DRMs is the possibility to use them as carriers for functional species within the MOF crystals. They can be readily doped with a variety of nanospecies, including metal, polymer or semiconductor nanoparticles, regardless of their chemical nature. This doping in turn allows for the synthesis of a novel class of active and adaptive MOF composites comprising a functional core surrounded by an ultra-porous framework; these composites are achieved without compromising the quality of the framework structure. These composites effectively combine the advantages of active nanoparticles with the porosity of the framework lattice. The method results in spatial control of the nanoparticle functionality inside the MOF crystal. Specifically, Pt and Pd nanoparticles have been chosen for the potential synergistic properties that can arise if combined with MOFs (for example, specific antitumor agents, highly selective catalysts, hydrogen storage systems) [28] , [29] , [30] ; luminescent CdSe-CdS-ZnS core-shell QDs and PTFE nanoparticles have also been embedded using the same method, foreseeing applications in the field of optics, optical sensing and drug storage/delivery (see the Methods section and Supplementary Figs S14–S19 ). The diverse nature of the encapsulated functional nanoparticles demonstrates the intrinsic versatility of the reported method. This new synthesis method is unlike the traditional procedure to synthesize host–guest MOF systems with heterogeneous species. The conventional route employs post-impregnation methods on grown crystals [14] , [31] . Here, we directly grow the MOF around the functionality. In this way, we avoid such undesirable effects as framework degradation and functionalization of the MOF exterior. Through the use of functionalized α-hopeite DRM seeds, a new generation of host–guest MOF systems, which possess a heart of active material surrounded by a molecular sieve, are envisaged. As an example of functional DRMs that harness MOF-5's specific filtering properties, we developed a light-emitting QDs/DRM/MOF-5 framework composite, which was demonstrated as a molecular sieve sensor. Using emission-quenching agents (thiols), it was shown that only thiols with a small enough molecular size could effectively diffuse through the framework and quench the emission of the functional QDs located in the crystals' cores. The real-time quenching tests demonstrate the validity of the proposed method for the fabrication of defect-free framework shells with an active core. The DRMs are a new tool to simultaneously tackle multiple issues that currently act as roadblocks to the implementation of MOF technology. Given the wide range of synthetic possibilities that the DRMs offer, new active MOF-based devices, such as sensors, micro-reactors, selective catalysts and other adaptive framework composites, can be now prepared in a straightforward, rapid and inexpensive manner. Materials All reactants were purchased from Sigma-Aldrich and used without any further purification. One-pot synthesis of DRMs encapsulated in MOF-5 A solution of 0.12 M zinc nitrate and 0.025 M terephthalic acid in DMF has been prepared by sonicating the precursors for 15 min. The main batch was then divided into 3.5 ml aliquots for MOF-5 growth experiments at different surfactant concentrations. Subsequently, amounts of Pluronic F-127 in the 0.05–0.4 g range were added to the vials, which were in turn sonicated for 15 min, at which time a colourless transparent solution was obtained. The sealed samples were then heated using an MRC dry bath incubator (Thermoline Scientific) at 95 °C preset temperature. The formation of DRMs was detected within the first minute of reaction. Depending on the concentration of surfactant, different densities of DRMs per unit volume were detected. The DRMs used for further experiments were extracted after 3 h using fritted glass filters (n. 1), and then re-dispersed in fresh DMF. Synthesis of MOF-5 in DEF All the DEF-based MOF-5 growing media used in the experiments with DRMs were prepared according to the same procedure described above, with the only difference being that DEF was used instead of DMF. The number of DRMs that effectively nucleate MOF-5 crystals can be maximized using a two-step heating process. This process can be performed on batches with the same precursor composition described above. The optimized procedure requires an initial heating step at 110 °C for 140 min, which is then followed by 20 h at 80 °C. Spatial control of MOF growth using DRMs on flat surfaces A drop of DRM suspension was deposited on an Al 2 O 3 or a silicon substrate, and the solvent was dried under vacuum to create a continuous bed of DRMs. The substrate was then broken in half by cutting it along the diameter of the circular DRM layer. One of the substrate halves was immersed in a typical DEF solution for MOF synthesis at 95 °C. After 12 h, MOF crystals were detected only in the region covered with DRMs. In accordance with the findings of Zacher et al . [32] , the bare alumina surface did not promote MOF formation. Spatial control of MOF growth using DRMs on patterned supports A concentrated suspension of DRMs in DMF was prepared by means of centrifugation and washing cycles, as described above. The lithographed substrates were fixed on an optical microscope stage under a ×10 magnification lens to allow for precise observation of the filling procedure. Filling was performed using a glass Pasteur pipette carefully drop-casting the microparticles directly onto the patterned areas. The procedure was repeated until the filling was complete. The substrates have then been dried under vacuum for 5 h, and eventually immersed into a standard DEF-based MOF-5 growing solution. The MOF-5 crystal growth was performed at 95 °C, according to the same procedure described above. Synthesis of DRMs functionalized with nanoparticles Functionalized DRMs have been prepared by adding nanoparticles directly into the typical solution used to synthesize DRMs. As an example, Pt and Pd functionalized DRMs were obtained by adding 0.7 ml of 5 μM noble metal colloidal solution to 3.5 ml of mother batch DRM solution; PTFE functionalized DRMs were synthesized by adding 8 mg of polymer nanoparticles into 3.5 ml of mother batch DRM solution; and QD-modified DRMs were prepared by adding 0.5 ml of 0.1 μM QD suspension in toluene to the standard 3.5 ml of mother batch DRM solution. The solutions have then been heated for 3 h at 100 °C and the functionalized DRMs collected and washed five times using fresh DMF; the DRMs were then inoculated into a fresh MOF-5 DEF mother batch solution. After 10–16 h MOF-5 crystals were collected and washed three times with DMF. Quenching test of QD suspensions using thiols Before performing the QDs/DRM/MOF-5 composites sieving test, the on/off sensitivity of the optical probe was verified. This verification was performed using standard emission quenching tests on free QDs suspended in anhydrous DEF. The selected QDs for the test have been yellow light-emitting (576 nm) CdSe-CdS-ZnS multi-shell nanoparticles synthesized according to a procedure adapted from JJ Li et al . [33] and reported in detail in the Supplementary Methods . The probe testing was performed with both static and time-resolved linear emission measurements. In a typical static test, 3 ml of a 1 μM QDs suspension were introduced into a quartz cuvette, which was placed inside the dark sampling chamber of a Varian Spectrofluorimeter (Varian). As shown in Supplementary Figure S20, an emission spectrum of the suspension in the 500–650 nm wavelength range was first recorded using a 365 nm excitation light. Separately, a quenching solution was prepared by dissolving the selected thiol in anhydrous DEF to obtain a 50 mM nominal concentration; this procedure was adopted for each of the three thiols selected for the experiment. After measuring the first emission spectrum of the QDs in DEF, 50 μl of the quenching solution were added to the QD suspension inside the cuvettes. Thiol concentration is in excess by several orders of magnitude compared with that usually used in QD emission quenching studies [21] , [34] , [35] ; this concentration ensures the reliability of the probe and fast emission quenching kinetics at room temperature. A second emission spectrum was then recorded 20 min after the injection. Quenching tests of QDs/DRM/MOF-5 composites using thiols A batch of DRMs functionalized with yellow QDs was used to nucleate MOF-5 crystals in DEF. The highly luminescent QDs/DRM/MOF-5 composites are shown in a digital photograph ( Supplementary Fig. S23a ). The presence of QDs embedded within the crystals is easily illustrated using a low power bench ultraviolet light. The crystals are cubic MOF-5 with an embedded QD functionalized DRM sitting in the middle of each crystal, as shown in the optical microscope image ( Supplementary Fig. S23b ). Immediately after the MOF-5 growth, the samples underwent a two-step washing process, consisting of four subsequent overnight solvent extractions with fresh and anhydrous DEF; the washing procedure was performed under a nitrogen atmosphere to minimize any contact with atmospheric moisture. All the quenching tests were performed on QDs/DRM/MOF-5 composites belonging to the same reaction batch. Three sealable quartz cuvettes were prepared for the emission measurements, and the amount of luminescent sample material for each cuvette was tailored to obtain comparable emission intensity at the beginning of each test. The crystals, sitting on the bottom of the quartz cuvette, were immersed in 1 ml of anhydrous DEF and kept under nitrogen flux for the duration of the test. A cyclic spectrum acquisition protocol was set up in the Spectrofluorimeter control software to automatically acquire an emission spectrum every 10 min. Thirty minutes after the acquisition was launched, a 100 μl quenching shot was injected dropwise into the sealed vial using a Hamilton syringe. How to cite this article: Falcaro, P. et al . A new method to position and functionalize metal-organic framework crystals. Nat. Commun. 2:237 doi: 10.1038/ncomms1234 (2011).